First-order coil-globule transition driven by vibrational entropy By shifting the balance between conformational entropy and internal energy, polymers modify their shape under external stimuli, such as changes in temperature. Prominent among such transformations is the coil-globule transition, whereby a polymer can switch from an entropy-dominated coil conformation to a globular one, governed by energy. The nature of the coil-globule transition has remained elusive, with evidence for both continuous and discontinuous transitions, with the two-state behaviour of proteins as an instance of the latter. Theoretical models mostly predict second-order transitions. Here we introduce a model that takes into consideration hitherto neglected features common to any polymer. We show that a first-order phase transition smoothly appears as a function of the model parameters. Our results can relieve part of the conflicts between theory and experiments in the field of protein folding, in the wake of recent studies tracing back the remarkable properties of proteins to basic polymer physics. The coil-globule transition (CGT) [1] is one of the most important phenomena exhibited by polymeric systems; polymers collapse into compact globules in a bad solvent, that is, a solvent that is unable to screen the mutual attraction between monomers, whereas they expand to coil-like conformations in a good solvent, where the only relevant interaction is the repulsive volume exclusion between monomers [2] . The CGT lies behind well-established technologies based on responsive polymers [3] , as well as emerging applications to drug delivery [4] and microfluidic devices and sensors [5] , and it sets the logical framework to understand protein folding [6] , possibly the most important natural occurrence of polymer collapse. Because of such widespread and crucial experimental and technological relevance, the CGT has been under careful theoretical scrutiny for the past three decades. In fact, there is a general agreement on the bad and good solvent sides of the transition. Instead, understanding the behaviour at the transition point represents a greater challenge. In his seminal work, de Gennes [7] , [8] built upon the approach of Flory [9] to describe the CGT as the transition of a tricritical magnetic system, inferring that it had to be a continuous transition. Although a large number of experiments have confirmed such prediction, there has also been evidence for discontinuous transitions [10] , [11] , [12] , findings that have been to date difficult to reconcile with the theory. Moreover, and more fundamentally from a conceptual point of view, proteins are known to undergo in most cases a two-state kind of transitions, where the folded (native in the biochemistry language) and the unfolded states coexist at the transition. This is very much akin to what is expected for discontinuous, first-order phase transitions, that are indeed characterized by phase coexistence. Although the special (non-random) heteropolymeric features of proteins have a crucial role in protein thermodynamics [13] , it must be noted that no simple protein model with designed sequence exhibits full-fledged coexistence at the transition. It becomes thus necessary to understand how the continuous transition predicted by de Gennes [7] , [8] can be turned into a discontinuous one as shown by proteins [6] , [14] , and whether it is possible to do so. Two paths have been previously proposed to that goal. In an early attempt [15] , [16] , and more recently in a paper by Doniach et al . [17] , polymers were endowed with a stiffness penalizing bent conformations, managing to elicit a new phase transition taking place within the globular phase and discriminating between amorphous and ordered globules. Such phase transition turned out to be similar to a first-order liquid–solid transition. Yet, the usual CGT retained its continuous nature. Only for very stiff polymers the collapse would take place directly toward ordered globules, thus changing the CGT order. A different strategy relies on the fine-tuning of the range of non-bonded interactions, so that within the globular phase, some rearrangements could lead from amorphous to ordered globules [18] . Again, this is a discontinuous transition that, for a carefully chosen interaction range, could pre-empt the CGT, which would otherwise remain continuous. Both these approaches, nonetheless, are unlikely to be relevant for synthetic polymers and proteins, that are very flexible [19] and equipped with interactions of many different types and ranges, unlikely to be so fine-tuned, as it is required for switching the order of the CGT. The approach we follow here is based instead on a critical analysis of traditional models of polymers. Taking into account hitherto neglected terms in the approximation of realistic Hamiltonians, we identify a single key parameter whose variation can result in a switch of the transition from continuous to discontinuous. Furthermore, we highlight how the subtle interplay between such parameter and the polymer length controls the emergence of the distinguishing features of first-order phase transitions, in particular phase coexistence. The self-interacting polymer model Polymers are made of monomers strung together in long chains. Monomers can be simple, as in polyethylene (one carbon atom with two side hydrogens), or complex, as amino acids in proteins. The covalent nature of the backbone interactions enforces almost fixed distances between consecutive monomers, whereas their mutual bending and torsional (dihedral) angles are restrained to discrete sets of values. For example, in polyethylene, the bond length is 0.153 nm, the angle between two bonds is about 112°, and three consecutive bonds are prevalently arranged in trans, gauche + or gauche − conformations [20] . As mentioned above, the interactions between non-consecutive monomers are governed by two contrasting terms: short-range repulsive volume exclusion, which forbids any two monomers to occupy the same region of space, and medium-range attractive forces such as hydrogen-bonds, hydrophobic and van der Waals interactions. Because of the tight constraints on monomer–monomer distances and relative angles, polymers mostly populate only a discrete set of conformations. These features are captured by a lattice description, where consecutive monomers occupy nearest-neighbour lattice sites and two monomers cannot lie at the same site. As a consequence, it is a deeply rooted belief that lattices can be used to explore the properties of real polymers [21] . In particular, by including an energy term that favours pairs of non-consecutive monomers to occupy neighbouring sites (usually called contacts), lattice polymers exhibit a CGT belonging to the same universality class as predicted by de Gennes [22] , [23] . The resulting model has been referred to as the Interacting Self-Avoiding Walk (ISAW). To improve upon the ISAW and identify the missing ingredients that may change the order of the CGT, it is necessary to review how the lattice embedding of real polymers is formally justified. The discrete set of conformations accessible to real polymers and captured by the lattice description are the inherent structures [24] (the minima) of a potential function that depends on the full set of coordinates in continuous space, , where is the three-dimensional position vector of the i -th monomer. The full partition function of a polymer of N beads is thus where Λ is the usual de Broglie thermal wavelength. If, in the spirit of a Gaussian approximation, only the dominant contribution of the set { γ }, corresponding to the conformations where attains its minimal value, is taken into account, equation (1) becomes The last term of equation (2) corresponds to the usual ISAW partition function; the energy is simply given by the number n ( γ ) of non-bonded contacts of conformation γ , each contributing an energy − ɛ (from here on, ɛ =1 and k B =1). Here we focus on the next term in the Gaussian approximation of equation (1), which accounts for the fluctuations of the polymer around the minima [25] Ĥ(γ) is the Hessian matrix of the potential evaluated at the minimum corresponding to conformation γ , and is the displacement of the i -th monomer from its equilibrium position in γ . Up to a multiplicative factor independent of the configuration, , (in the minima six eigenvalues vanish, corresponding to rigid rotations and translations). As − k B T ln[ w ( γ )] is the vibrational free energy associated with conformation γ , and the internal energy is trivially 3 Nk B T /2 for all conformations, w ( γ ) is seen to embody the effects of vibrational entropy of conformation γ . In our potential energy, the inherent structures correspond to conformations that can be embedded on the tetrahedral lattice. With this choice, bending angles between consecutive bonds have an equilibrium value of , whereas four-body dihedral angles can take the three different equilibrium values . The minimum of the contact energy between non-consecutive monomers is set at a distance, which is precisely the lattice spacing l ( l =1 henceforth). The complete potential then reads where k bb , k θ , k ψ t , g and k are the stiffness constants of the bonds between consecutive monomers, of the angles between consecutive triplets, of the dihedral angles between consecutive quadruplets and of the non-bonded nearest-neighbour forces, respectively. The parameter k ψ t , g further distinguishes between trans and gauche conformations (see Methods ). The contact matrix Δ i , j is equal to 1 if non-consecutive ( j ≠ i ±1) monomers i and j are nearest neighbours, and it is zero otherwise. The Hessian matrix of the energy function (equation (4)) is then obtained after expressing the bending and dihedral angles using Cartesian coordinates and expanding to second order in the displacements . We have then compared the behaviour of the traditional ISAW equation (2) model and of the present scheme, that we have termed, for brevity, Vibrating ISAW, henceforth VISAW, equation (3). Thermodynamics The thermodynamic behaviour of the ISAW model confirms that the associated CGT is continuous in three dimensions, as already found previously [22] . The microcanonical entropy is , where is the number of conformations with a given energy E , and its derivative with respect to E yields the inverse temperature, β =1/ T = dS ( E )/ dE . 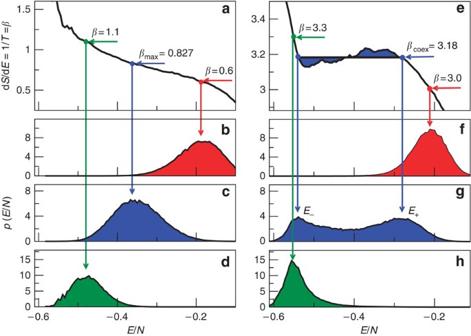Figure 1: Model thermodynamics. The microcanonical behaviour of polymers according to the ISAW (left column) and VISAW (right column) forN=180. (a) The derivative of the entropy with respect to the energy, proportional to the number of contacts, corresponds to the inverse temperatureβ=1/T. The slope is always negative, corresponding to a physical positive specific heat; the energy probability distribution is sampled at temperatures (b) higher than, (c) equal to and (d) lower than the temperature of the maximum of the specific heatTmax, and in all cases it is found to be unimodal. (e) A positive slope corresponds to a microcanonical negative specific heat, which is not physical in the canonical ensemble and needs, therefore, the Maxwell construction to be avoided; the energy probability distribution at temperatures (f) higher than and (h) lower thanTcoexare unimodal, whereas at a temperature equal toTcoex(g) the coexistence of two phases of low and high energy is marked by the presence of two distinct peaks atE−andE+. Figure 1a–d show that β is a monotonously decreasing function of the energy, with no signs of phase coexistence. The picture changes dramatically in the VISAW model. Consistently with our canonical simulations (see Methods ), we define the VISAW microcanonical entropy as , where the sum runs over all the conformations γ characterized by an energy E . As for the ISAW, here E refers to the contact part only of the energy. Figure 1e–h reveal that the derivative of S ( E ) is no longer monotonic when vibrations are included in the picture. The region where β grows with E , which would correspond to a negative microcanonical specific heat, is canonically forbidden and is one of the hallmarks of a discontinuous transition with coexistence between two different phases [26] , [27] , [28] . The coexistence temperature can be extracted from the β ( E ) curve using the customary Maxwell construction; this value β coex ≃ 3.18 agrees well with the temperature of the (canonical) specific heat maximum β max =3.20(2). Figure 1: Model thermodynamics. The microcanonical behaviour of polymers according to the ISAW (left column) and VISAW (right column) for N =180. ( a ) The derivative of the entropy with respect to the energy, proportional to the number of contacts, corresponds to the inverse temperature β =1/ T . The slope is always negative, corresponding to a physical positive specific heat; the energy probability distribution is sampled at temperatures ( b ) higher than, ( c ) equal to and ( d ) lower than the temperature of the maximum of the specific heat T max , and in all cases it is found to be unimodal. ( e ) A positive slope corresponds to a microcanonical negative specific heat, which is not physical in the canonical ensemble and needs, therefore, the Maxwell construction to be avoided; the energy probability distribution at temperatures ( f ) higher than and ( h ) lower than T coex are unimodal, whereas at a temperature equal to T coex ( g ) the coexistence of two phases of low and high energy is marked by the presence of two distinct peaks at E − and E + . Full size image The difference between Fig. 1a and e , in particular, points to the vibrational entropy as the culprit for the change in the order of the transition. As a matter of fact, in the context of solid–solid transformations, it had already been observed that the specific heat is enhanced at the transition if the high-temperature phase is softer, that is, richer in low-frequency vibrational modes [29] , than the low-temperature one. In the present case, the scenario is even more dramatic because the coil and globule phases are completely different from a topological point of view; coils are low-dimensional, typically soft structures, whereas globules are higher-dimensional and stiffer conformations. More precisely, the difference in rigidity between coil and globule conformations is controlled by the elastic constant k associated with non-bonded interactions. Coil conformations, featuring few contacts, are characterized by vibrational spectra rather insensitive to changes in k ( Fig. 2a ). By converse, the spectra of globular conformations crucially depend on k ; for k =0, only backbone potential terms (bond-length, bending and torsional angles) are present, so that all conformations have a vibrational spectrum akin to those of coils ( Fig. 2b ); as k increases, the elastic terms transverse to the backbone become progressively more important, making the spectra more similar to what is expected for a compact solid, with a dramatic depletion of low-frequency modes, the ones that contribute the most to the entropy. 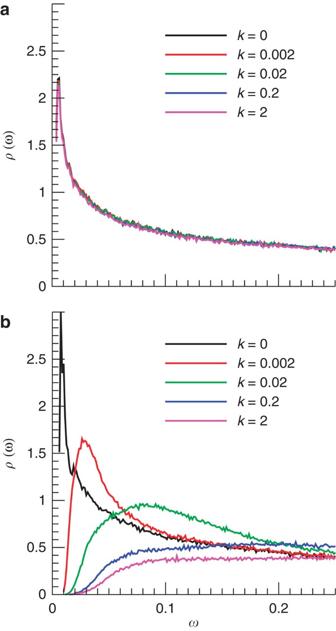Figure 2: Vibrational density of states. Low-frequency part of the density of vibrational states as a function of the frequency(theλs are the eigenvalues of the Hessian matrix) for polymers of lengthN=100 and for various values of the contact stiffness parameterk: (a) coil-like conformations (5 contacts); (b) compact conformations (number of contacts between 52 and 59). The absence of a relevant dependence onkfor coil conformations contrasts with the dramatic effect thatkhas on compact conformations. Figure 2: Vibrational density of states. Low-frequency part of the density of vibrational states as a function of the frequency (the λ s are the eigenvalues of the Hessian matrix) for polymers of length N =100 and for various values of the contact stiffness parameter k : ( a ) coil-like conformations (5 contacts); ( b ) compact conformations (number of contacts between 52 and 59). The absence of a relevant dependence on k for coil conformations contrasts with the dramatic effect that k has on compact conformations. Full size image Three consequences proceed from the above argument. First, the discontinuous nature of the phase transition should be magnified by increasing values of k , as the depletion of low-frequency modes becomes more pronounced ( Fig. 2b ). Second, the discontinuous nature of the phase transition should equally become more evident for increasing values of the polymer length N , at constant values of k , because the vibrational modes of longer polymers are progressively softer, hence the low-frequency region more populated and thus the depletion induced by k ≠0 more relevant. Third, for k =0, the ISAW and the VISAW should fall in the same universality class, because the entropy weight is roughly the same for coil and globule conformations ( Fig. 2a,b for k =0), and is, to a good approximation, a simple multiplicative constant for the partition function. To prove the above inferences, we have analysed the energy probability distribution in these three scenarios. For a fixed length ( N =180), the histogram does indeed evolve from single to two-state as k increases ( Fig. 3a–d ). The evolution of the density of states for a fixed k and growing lengths ( Fig. 3e–h ) reveals that phase coexistence emerges as the length is increased, as argued above. To obtain a complete picture, we finally inspected how the density of states changes with length as k =0; no coexistence appears, and the energy histogram approaches, as argued above, one of the traditional tricritical model, which thus defines the universality class for k =0 ( Fig. 3i–l ). 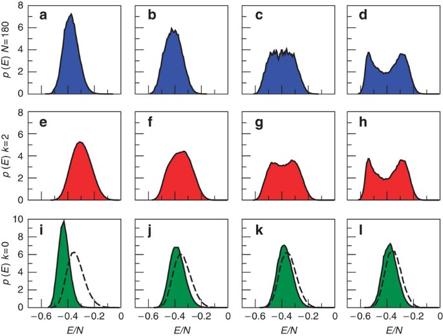Figure 3: Evolution of the energy probability distribution of the VISAW. The first row portrays the evolution of the energy (per monomer) probability distribution for a fixed polymer length,N=180, and varying values ofk(panela:k=0,b: 0.02,c: 0.2 andd: 2). As it can be clearly seen, the distribution progressively broadens until two peaks become clearly discernible, signalling phase coexistence. The second row reports the evolution of the distribution for a fixed value ofk(k=2) and progressively longer polymers (panele:N=50,f: 100,g: 140 andh: 180). As for the first row, the distribution becomes broader and, eventually, characterized by two peaks. The behaviour of the VISAW model fork=0 and increasing lengths (i–l, same length sequence as for the second row) approaches the one of the standard ISAW model (dashed line), suggesting that the ISAW model and the VISAW model fork=0 belong to the same universality class. Figure 3: Evolution of the energy probability distribution of the VISAW. The first row portrays the evolution of the energy (per monomer) probability distribution for a fixed polymer length, N =180, and varying values of k (panel a : k =0, b : 0.02, c : 0.2 and d : 2). As it can be clearly seen, the distribution progressively broadens until two peaks become clearly discernible, signalling phase coexistence. The second row reports the evolution of the distribution for a fixed value of k ( k =2) and progressively longer polymers (panel e : N =50, f : 100, g : 140 and h : 180). As for the first row, the distribution becomes broader and, eventually, characterized by two peaks. The behaviour of the VISAW model for k =0 and increasing lengths ( i – l , same length sequence as for the second row) approaches the one of the standard ISAW model (dashed line), suggesting that the ISAW model and the VISAW model for k =0 belong to the same universality class. Full size image Scaling properties at the transition The non-analytic part of the extensive free energy of self-interacting polymers in the proximity of the transition is, by scaling arguments [30] , of the form where t =( T − T C )/ T C is the reduced temperature ( T C being the transition temperature) and φ is the crossover exponent. Thus, the specific heat, which is the second derivative of the free energy per monomer with respect to temperature, scales at the transition ( t =0) as C v ∼ N 2 φ −1 . As a consequence of the mean-field nature of tricritical transitions in three dimensions, φ =1/2, implying that C v ∼ const (with expected logarithmic corrections) [8] , [23] , [31] . By converse, in the presence of a first-order phase transition, the crossover exponent is φ =1 and C v ∼ N , by standard finite-size arguments [32] , [33] . Interestingly, the inverse relation t ∼ 1/ N (consistent with φ =1) has been observed for a collection of proteins of various lengths, strengthening the case for a first-order-like protein-folding transition [34] . Our simulations confirm such predictions ( Fig. 4a ); the specific heat of the ISAW model barely grows with an effective crossover exponent φ =0.56, compatible with the expected φ =1/2 dressed by logarithmic corrections and/or finite-size effects. When instead fluctuations around the energy minima are taken into account, for k =2 the specific heat grows more than linearly with N . As the extensivity of the energy sets φ =1 as the upper bound for the crossover exponent, we interpret superlinearity as a transient behaviour due to the increasing separation of the two energy peaks corresponding to the coexisting phases (see Figs 1g and 3e–h ). Once the distance between the two peaks has stabilized, the crossover exponent attains its asymptotic value φ =1. Calorimetry, thus, confirms the discontinuous nature of the transition of the present model. 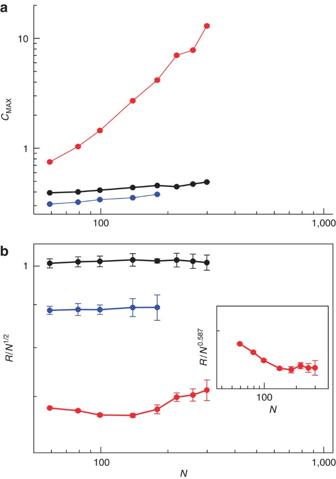Figure 4: Scaling properties at the coil-globule transition. (a) Log–log plot of the maximum of the specific heat,CMAXas a function of the polymer lengthNfor the ISAW model (black circles) and for the VISAW model in the two casesk=0 (blue circles) andk=2 (red circles). The VISAW-specific heat has been reduced by a factor to be plotted with the much lower one of the ISAW without compressing too much the latter. (b) Log–log plot of the ratio of the average radius of gyration,R, to the expected ideal scaling behaviour,N1/2, as a function of the polymer length. The data for the ISAW and VISAW (k=0) models have been taken at the transition point, identified as the temperatureTCwhere the curvesR(T)/N1/2intersect, rather than as the temperature of the maximum of the specific heat, which is affected by considerable finite size effects. Importantly, in both cases, a temperatureTCis well identified from the data (not shown). In the case of the VISAW (k=2), the data have been taken at the temperature of the maximum of the specific heat, as in this case no clear temperature can be found where the curvesR(T)/N1/2intersect, and because the data show, especially for longer polymers, that the transition temperature identified using the Maxwell construction (Fig. 1e) coincides with the one of the maximum of the specific heat. The inset shows the behaviour ofR(N)0.587as a function of polymer length to highlight that for longer lengths VISAW polymers behave as self-avoiding chains. Data keys in panelbare the same as in panela. Figure 4: Scaling properties at the coil-globule transition. ( a ) Log–log plot of the maximum of the specific heat, C MAX as a function of the polymer length N for the ISAW model (black circles) and for the VISAW model in the two cases k =0 (blue circles) and k =2 (red circles). The VISAW-specific heat has been reduced by a factor to be plotted with the much lower one of the ISAW without compressing too much the latter. ( b ) Log–log plot of the ratio of the average radius of gyration, R , to the expected ideal scaling behaviour, N 1/2 , as a function of the polymer length. The data for the ISAW and VISAW ( k =0) models have been taken at the transition point, identified as the temperature T C where the curves R ( T )/ N 1/2 intersect, rather than as the temperature of the maximum of the specific heat, which is affected by considerable finite size effects. Importantly, in both cases, a temperature T C is well identified from the data (not shown). In the case of the VISAW ( k =2), the data have been taken at the temperature of the maximum of the specific heat, as in this case no clear temperature can be found where the curves R ( T )/ N 1/2 intersect, and because the data show, especially for longer polymers, that the transition temperature identified using the Maxwell construction ( Fig. 1e ) coincides with the one of the maximum of the specific heat. The inset shows the behaviour of R ( N ) 0.587 as a function of polymer length to highlight that for longer lengths VISAW polymers behave as self-avoiding chains. Data keys in panel b are the same as in panel a . Full size image The metric properties of polymers at the transition are also of fundamental interest. Polymers below the transition are compact globules and their radius of gyration R scales with their length as R ∼ N 1/3 . Much above the transition temperature, the only relevant inter-monomer interaction is excluded volume and R ∼ N ν SAW , where ν SAW ≃ 0.587 is the exponent of three-dimensional self-avoiding walks [35] . Once again, due to the tricritical nature of the transition, characterized by mean-field values of the exponents in three dimensions, at the transition point ISAW polymers behave as ideal chains, with the radius of gyration R scaling as the square root of the number of monomers ( R ∼ N 1/2 ). The behaviour of R / N 1/2 as a function of N at the ISAW CGT transition is shown in Fig. 4b , confirming the theoretical predictions. Two regimes are instead clearly discernible in the metric properties of the VISAW model at the coexistence temperature; polymers of small length ( N ≤100) behave as random coils ( R ∼ N 1/2 ), whereas longer polymers ( N ≥140) scale as SAWs (inset in Fig. 4b ). These results are a consequence of the discontinuous nature of the transition, where no divergences are expected. Indeed, the critical behaviour of the ISAW model conforms to the usual scaling at continuous transitions; the ideal metric properties encompass a number of monomers that scales as t −1/ φ , as posited by equation (5), diverging as the whole polymer is taken up at t →0. By converse, at a discontinuous transition, the critical region remains of finite size, so that the ideal behaviour that we observe can extend only up to finite lengths, and must cross over to the dominant non-critical scaling, which in the present case is represented by the self-avoiding exponent ν ≃ 0.587 (inset of Fig. 4b ). To provide a more complete picture, we have also analysed the scaling properties of the VISAW model for k =0 ( Fig. 4a,b ), confirming that in the absence of vibrations of non-bonded contacts, VISAW polymers remain in the ISAW universality class. Ever since de Gennes showed that, for the ISAW model, the CGT is continuous, identifying the features capable of changing its order has remained one of the major challenges in polymer physics. In the years, several different modifications have been proposed, such as switching from flexible to semi-flexible polymers [15] , [16] , [17] , or suitably tuning the range of the non-bonded attractive interactions [18] . These previous attempts have never really succeeded in changing the order of the CGT, which is instead simply pre-empted by a first-order transition under special conditions, such as strongly reduced flexibility of the chain backbone or very narrow-range interactions. As such scenarios do not really apply to proteins and synthetic polymers, whether any basic polymer model could produce the desired discontinuous transition has remained an unanswered issue. The VISAW model that we presented here is a natural generalization of the ISAW, stemming from basic considerations about the structure of a realistic potential compatible with the ISAW approximations. The inclusion of fluctuations around inherent structures in the calculation of the partition function is coherent with modern developments in condensed matter physics [25] and provides a clearer picture of the CGT. The change in the order of the transition is brought about by the force constant k of non-bonded contacts, because of its depleting effect of low-frequency modes for globular conformations. It is crucial here to stress that it is not the absolute flexibility of the polymers that determines the transition order change, but rather the softness difference between globule and coil conformations. Our results also shed light on some difficulties that have hindered the assessment of the CGT order from the experimental point of view, and on the problems at reconciling the two-state behaviour of proteins with fundamental polymer physics. Indeed, very soft, non-bonded contacts (small k values in the VISAW model) would not manifest the discontinuity of the transition if not for extremely long polymers. By converse, stiff contacts (high k values) would induce phase coexistence for shorter polymers. In this respect, proteins stand out because the interactions between adjacent amino acids include, most of the time, hydrogen-bond interactions as in secondary structures ( α -helices and β -sheets). The hydrogen bond is rather rigid, as captured by coarse-grained models where its stiffness can be up to tens of times larger than for van der Waals or hydrophobic interactions [36] . As a consequence, at variance with other polymers with softer interaction, such as polyethylene, polymethylene or polystyrene, proteins might be more likely to exhibit two-state behaviour already at intermediate lengths. At the same time, the limited length of proteins clearly hinders the possibility to unambiguously distinguish discontinuous from continuous transitions [6] , [37] . Moreover, it is important to recall that the non-random heterogeneity of the amino acid sequence is likely to contribute to the sharpness of the transition in proteins [13] . The VISAW model that we have introduced here contributes thus to a recent emerging scenario where salient features of proteins, such as the two-state behaviour and the presence of secondary structures, would be attributed to previously unexplored general properties of simpler homopolymers [38] , [39] . The results shown here inevitably raise several issues. First and foremost, it is crucial to discuss the relations of the present model with other approaches that have been used in the past to study the CGT. In particular, both lattice and off-lattice models have lent support to the continuous transition framework. In a previous section, it has been shown how the VISAW model builds upon the usual approximations leading to lattice models, pushing them one step further toward lattice polymers closer to the real ones. The connection with off-lattice schemes is instead more delicate. Indeed, most off-lattice approaches describe polymers as freely jointed chains of beads, with no bending and, most importantly, no torsional potentials [23] , [40] . A polymer whose backbone is described by a potential similar to the one of equation (4) can be considered as fully flexible in the following scenarios: either some re-scaling is implicitly invoked, such that the connection between consecutive beads actually captures several chemical monomers that are in a random coil conformation, or the energy barrier between torsional minima is much lower than the thermal energy at the CGT, in which case polymers do not feel any torsional restriction. Neither assumption, yet, is likely to apply to real polymers; the re-scaling procedure leading to a freely jointed description cannot be applied equally well to the coil and to the globule phases, as they are conformationally different both at the global and local scales; as well, it has been shown that realistic torsional potentials do strongly confine conformations at room temperature [41] , [42] , which is close to the CGT for real polymers, implying that the barriers between trans and gauche ± conformations are significantly larger than the thermal energy. As a consequence, we argue that a flexible, torsion-free polymer model is not necessarily a good model to describe the CGT of real polymers. Furthermore, it is not easy to draw conclusions about the connections between lattice VISAW and off-lattice torsion-free polymers, as the latter cannot be recovered as a limit of the former. Rather a full-fledged off-lattice study would be needed, with the energy barrier between torsional minima as an extra parameter. The present work has also some more theoretical, and in some sense fundamental, implications. As k =0 still belongs to the ISAW universality class but k≠ 0 does not, our generalization has actually introduced a new parameter that is relevant, in a renormalization group perspective, because it leads away from the usual tricritical point. Further simulations for small values of k , thus close to the ISAW CGT, could also uncover the scaling relation between k , t and N , leading to a free energy of the form with φ t the usual crossover exponent. Unfortunately, the heavy computational costs implied by the need to diagonalize the Hessian matrix at each Monte-Carlo step is presently hindering our capability to analyse, with reliable statistics, the large span of lengths that would be necessary to assess such subtle scaling features. This, as many other analyses, will be needed in the future to fully understand the properties of this new model and to unveil its connections with the behaviour of real polymers and proteins. Details of the model In this work, we adopted non-dimensional units. In particular, the energy of non-bonded monomer contacts is ɛ =1 and the Boltzmann constant k B =1. Temperature is expressed in units of ɛ / k B . The lattice spacing is set to l =1, and the stiffness constants of the potential equation (4) are expressed in units of energy. The stiffness constants of the elastic potential equation (4) are set to k bb =150, k θ =1, k ψ t = 1 and k ψ g = 0.6. The non-bonded interaction constant k is varied in the range (0,2). The stiffness of the bond between two consecutive monomer pairs, k bb , is much larger than the others, consistently with other coarse-grained off-lattice force fields [36] , [43] , [44] where the bond is rigid ( k bb =∞). This choice reflects the almost fixed length of a covalent bond. The ratio between the trans ( k ψ t ) and gauche ( k ψ g ) stiffness constants is such that the eigenvalues of the corresponding Hessian sub-matrices are equal. In this way the trans and the gauche direction are individually associated with the same weight and we avoid introducing any chain semi-flexibility that was already treated in previous models [15] , [16] , [17] . The sum over consecutive quadruplets (third term of equation (4)) can be expressed more explicitely as three sums over the trans, gauche + and gauche − quadruplets: where each quadratic term corresponds to the second-order expansion of a potential that can be written as [45] with the a k coefficients chosen so that V ( ψ i +3, i ) has three minima of the same value in ψ i +3, i =π, ±π/3 with second derivative . The number of a k coefficients depends then on the number of further conditions that are imposed on V ( ψ i +3, i ). Details of the simulations and of data analysis The model was investigated on the tetrahedral lattice by means of dynamic Monte Carlo with Pivot moves [46] , [47] . Each new proposed configuration ( γ new ) is accepted, if self-avoiding, with probability The Multiple Histogram Method technique [48] was used to merge data obtained from simulations at different temperatures and fixed length. The error bars were estimated with the bootstrap method. The derivative of the microcanonical entropy β =d S ( E )/d E ( Fig. 1 ) was calculated by means of a low-noise Lanczos differentiator [49] . How to cite this article : Maffi, C. et al . First-order coil-globule transition driven by vibrational entropy. Nat. Commun. 3:1065 doi: 10.1038/ncomms2055 (2012).